Sub-resolution lipid domains exist in the plasma membrane and regulate protein diffusion and distribution Lipid microdomains are postulated to regulate many membrane-associated processes but have remained highly controversial. Here we provide the first direct evidence that the plasma membrane of intact, live cells is comprised of a sub-resolution mixture of approximately 76% ordered and 24% disordered lipid domains, which correspond to liquid-ordered and -disordered model membranes. These measurements were based on the unmixing of fluorescence lifetime decays (phasor analysis) obtained from environmentally sensitive membrane dyes that report the degree of lipid packing. Using the transmembrane protein Linker for Activation of T cells (LAT) as an example, we demonstrate that association with ordered domains retarded LAT diffusion and decreased clustering in meso-scaled protein domains as analysed by super-resolution microscopy. Our data therefore propose a membrane model in which the majority of the plasma membrane is covered by cholesterol-dependent, ordered lipid domains that contribute to the non-random distribution and diffusion of membrane constituents. The lipid raft hypothesis postulates the existence of cholesterol (Chol)-enriched, ordered-phase lipid domains in cell membranes [1] . As demonstrated for model membranes [2] , liposomes reconstituted from cell lipids [3] and plasma membrane vesicles and spheres [4] , [5] , [6] , the lipid bilayer can separate into two distinct liquid phases known as the liquid-ordered and -disordered phases [2] . Membrane proteins with a differential affinity for lipid domains can therefore be laterally sorted [7] . However, large-scale lipid-phase separation has not been observed in native cell membranes, raising the question whether stable lipid rafts exist in this environment [8] , [9] , [10] . It has therefore been suggested that lipid rafts must be below the resolution of optical microscopes and/or transient in nature [1] . Analysis of the localization [11] , oligomerization [12] , [13] , transient confinement [14] and diffusion properties [15] , [16] of membrane proteins have been interpreted in this context [1] , although other explanations have also been provided, such as nanoclusters and proteins islands [17] , confinements by the actin cytoskeleton [18] and membrane topography [19] . The difficulties in providing direct evidence for lipid domains are twofold. First, lipid organization is best observed in live cells because fixation can induce artifacts [20] , but the resolution of optical microscopy is limited. Second, the assumption has to be made that fluorescent lipid analogues behave identically to native lipids. Here we use common membrane dyes that report lipid packing of the surrounding bilayer in model and cell membranes [6] , [21] , [22] : Laurdan and di-4-ANEPPDHQ. Laurdan, a derivative of Prodan, displays a spectral red shift in emission between the liquid-ordered and -disordered phases, as well as a shortening of its fluorescence lifetime. These shifts are due to the differential penetration of polar water molecules into the non-polar bilayer in the two phases. The probe di-4-ANEPPDHQ shows similar environmental sensitivity to Laurdan [23] , [24] . In numerous previous studies, the spectral shifts were quantified in a normalized intensity ratio, known as generalized polarization (GP) [22] . Here we analysed the fluorescence lifetime shifts with the phasor approach to fluorescence lifetime imaging microscopy (FLIM) data, which unmixes multi-exponential lifetime decay components of the fluorescence signal in each pixel [25] , [26] . The phasor approach is a model-free assessment of the composition of fluorescence decays without any a priori assumptions of the number of decay components. When applied to FLIM data of membrane-order sensing dyes, it is therefore possible to evaluate in an unbiased manner whether cellular membranes have a homogenous lipid order or are mixtures of different lipid-order microenvironments in each pixel. Phase separation in model and cell membranes To demonstrate the suitability of the Laurdan FLIM/phasor approach, we first recorded FLIM data from Laurdan-stained lipid vesicles. The data were converted into the frequency domain and plotted on a phasor plot [26] , which is a vector-like two-dimensional histogram of sine-cosine transformed lifetime decays from each pixel ( Fig. 1a ). If the membrane dye exhibits single-exponential lifetimes from homogenous lipid environments, the values must lie on the universal circle, whereas multi-exponential decays from a mixture of two or more of these lipid environments lie inside the circle. For a double-exponential decay from two single-exponential profiles, the data must lie on a chord intercepting the universal circle at the individual two lifetimes ( Fig. 1a ). Laurdan’s fluorescence decay (when excited at 405 nm and detected through a 430 nm long-pass filter) from homogenous membranes composed of 100% dioleoylphosphatidylcholine (DOPC), and of 70% palmitoylsphingomyelin (SM) and 30% Chol (SM:Chol 7:3), which reside in the liquid-disordered and -ordered phases, respectively [27] , lie on or near to the universal circle ( Fig. 1b ), indicating that the decays were close to single exponential under these conditions. Data from a lipid mixture (SM:DOPC:Chol 1:1:1) that undergoes phase separation between 20 and 30 °C were close to the chord connecting the positions of the pure liquid-ordered and -disordered phases at low temperature, indicating the co-existence of lipid phases. At high temperature, the signal is mono-exponential, indicating a homogenous phase of intermediate order ( Fig. 1c ). 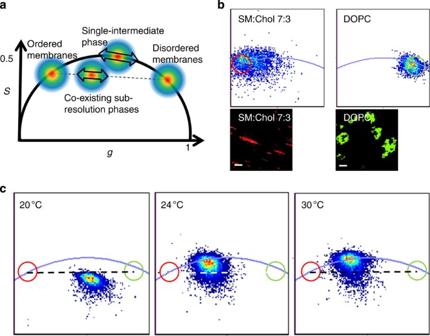Figure 1: Phasor plots of the order-sensitive membrane dye Laurdan in model bilayers. Experimental FLIM data of Laurdan-stained-membranes were obtained by time-correlated single-photon counting and plotted as phasor plots. (a) Schematic representation of a phasor plot. FLIM data of Laurdan (excitation 405 nm, emission >430 nm) located in homogeneous lipid environments have single-exponential fluorescence decays and therefore lie on the universal circle (bold line). Longer-to-shorter lifetimes corresponding to more ordered-to-disordered membranes travel clockwise along the universal circle. Laurdan’s lifetime decays from a heterogeneous lipid environment of two immiscible lipid phases are bi-exponential and lie on a chord connecting the two individual decay components (dashed line). The position along the chord indicates the fraction of the fluorescence originating from each phase. (b) Phasor plots and grey-scale images of artificial membranes composed of ordered bilayers (SM:Chol 1:1) and disordered bilayers (DOPC). All the phasor data points lie close to the universal circle indicating mono-exponential lifetimes and, hence, homogeneous lipid environments. Highlighted regions in the phasor plot correspond to long-lifetime decays emanating exclusively from ordered membranes (red circle and pixels) and short-lifetime decays, which all originate from disordered bilayers (green circle and pixels). Scale bar, 10 μm. (c) Phasor plots from a ternary mixture of SM:DOPC:Chol 1:1:1, which show predominately double-exponential decays on the cord (dash line) and therefore phase separation of the two pure phases at 20°C; and mono-exponential decays on the universal circle corresponding to an intermediate, homogeneous phase at 24°C and 30°C. Data are from one of the six representative experiments. Figure 1: Phasor plots of the order-sensitive membrane dye Laurdan in model bilayers. Experimental FLIM data of Laurdan-stained-membranes were obtained by time-correlated single-photon counting and plotted as phasor plots. ( a ) Schematic representation of a phasor plot. FLIM data of Laurdan (excitation 405 nm, emission >430 nm) located in homogeneous lipid environments have single-exponential fluorescence decays and therefore lie on the universal circle (bold line). Longer-to-shorter lifetimes corresponding to more ordered-to-disordered membranes travel clockwise along the universal circle. Laurdan’s lifetime decays from a heterogeneous lipid environment of two immiscible lipid phases are bi-exponential and lie on a chord connecting the two individual decay components (dashed line). The position along the chord indicates the fraction of the fluorescence originating from each phase. ( b ) Phasor plots and grey-scale images of artificial membranes composed of ordered bilayers (SM:Chol 1:1) and disordered bilayers (DOPC). All the phasor data points lie close to the universal circle indicating mono-exponential lifetimes and, hence, homogeneous lipid environments. Highlighted regions in the phasor plot correspond to long-lifetime decays emanating exclusively from ordered membranes (red circle and pixels) and short-lifetime decays, which all originate from disordered bilayers (green circle and pixels). Scale bar, 10 μm. ( c ) Phasor plots from a ternary mixture of SM:DOPC:Chol 1:1:1, which show predominately double-exponential decays on the cord (dash line) and therefore phase separation of the two pure phases at 20°C; and mono-exponential decays on the universal circle corresponding to an intermediate, homogeneous phase at 24°C and 30°C. Data are from one of the six representative experiments. Full size image We next imaged live HeLa cells with a confocal FLIM setup at a focal plane where both the plasma membrane and intracellular membranes were visible (an equatorial confocal section, Fig. 2 ). The lifetime values of Laurdan and di-4-ANEPPDHQ obtained from these images fell on the chord connecting the pure liquid-ordered (red) and -disordered (green) phases ( Fig. 2a , Supplementary Fig. S1 ). We quantified the alignment of Laurdan FLIM signals with the chord by extracting the g and S coordinates of the centre of the distribution of data points that correspond to pure liquid-ordered phases, -disordered phases, the plasma membrane and intracellular membrane. These four coordinates can be fitted to a straight line with an R 2 =0.9003. This strongly indicates that in cell membranes, order-sensitive dyes exhibited a double-exponential decay representing two distinct lipid phases, and not a homogenous phase of intermediate order. Thus, cell membranes are a mixture of two immiscible lipid environments corresponding to the two classic liquid-ordered and -disordered phases that have been observed in artificial membranes. This is the first direct evidence that two phases co-exist on sub-resolution length scales in native cell membranes, despite the absence of large, microscopically visible lipid domains. 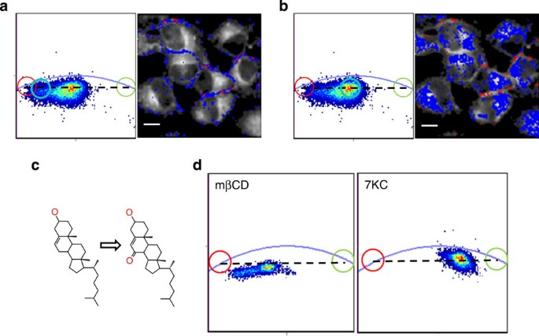Figure 2: FLIM phasor analysis of Laurdan in live HeLa cells. Live HeLa cells were labelled with Laurdan (5 μM, 30 min) and lifetime images of confocal equatorial section obtained at room temperature. In the phasor plots, intercepts of the cord (dashed lines) with the universal circle are marked by red and green circles that correspond to pure ordered and disordered phases, respectively. (a,b) Region-of-interest (blue circle) in the phasor plot that correspond to the plasma membrane (a) and intracellular membranes (b) as highlighted by blue pixels in the original image, mark the cord at ordered:disordered mixtures of 80:20 (a) and 47:53 (b), respectively. Scale bar, 10 μm. (c) Structure of cholesterol and 7-ketocholesterol. (d) Phasor data from HeLa cells treated with 5 mM mβCD for 20 min or incubated with 25 μM 7KC complexed to mβCD for 30 min. Data are representative of six cells. Figure 2: FLIM phasor analysis of Laurdan in live HeLa cells. Live HeLa cells were labelled with Laurdan (5 μM, 30 min) and lifetime images of confocal equatorial section obtained at room temperature. In the phasor plots, intercepts of the cord (dashed lines) with the universal circle are marked by red and green circles that correspond to pure ordered and disordered phases, respectively. ( a , b ) Region-of-interest (blue circle) in the phasor plot that correspond to the plasma membrane ( a ) and intracellular membranes ( b ) as highlighted by blue pixels in the original image, mark the cord at ordered:disordered mixtures of 80:20 ( a ) and 47:53 ( b ), respectively. Scale bar, 10 μm. ( c ) Structure of cholesterol and 7-ketocholesterol. ( d ) Phasor data from HeLa cells treated with 5 mM mβCD for 20 min or incubated with 25 μM 7KC complexed to mβCD for 30 min. Data are representative of six cells. Full size image When we selected a region-of-interest (blue circle, Fig. 2a ) in the phasor plot and marked the pixels from which those signals were derived in the cell image (blue pixels in Fig. 2a ), we observed that the centre of the region-of-interest that corresponds to the plasma membrane ( Fig. 2a ) was at a position 76±6% ( n =19 cells) along the chord that connects pure ordered-phase membranes (100%) and disordered-phase membranes (0%). This means that for the plasma membrane, on average 76% of detected photons derived from ordered-phase membranes. As Laurdan partitions approximately equally between the two phases [6] and assuming a similar quantum yield, the data demonstrate that the majority of the plasma membrane resides in the ordered phase. We reached a similar conclusion when sparsely seeded cells were imaged at higher magnification ( Supplementary Fig. S2 ) or when the basal plasma membrane adjacent to the glass coverslip was analysed ( Supplementary Fig. S3 ). To achieve such high coverage, ordered domains either have a large range of sizes to enable close packing of domains or disordered domains exist in a continuous, percolating liquid-ordered phase. This is contrary to classical models, although similar models were reported previously. The first model was proposed for rabbit red blood cells with ordered domains ranging from 25 to 300 nm in diameter [28] , whereas the later conclusion was made for the apical membranes of polarized epithelial cells [29] and plasma membrane-derived vesicles [30] . In contrast, intracellular membranes contain only 49±16% ( n =19 cells) ordered membranes ( Fig. 2b ). Next, we treated the cells with methyl-β-cyclodextrin (mβCD), which removes cellular Chol, or 7-ketocholesterol (7KC), which reduces membrane order [31] ( Fig. 2d ). As expected, mβCD treatment lowered the percentage of the fluorescence derived from the ordered phase from 76±6% to 70±3% ( P <0.05), indicating that the ordered-phase domains are indeed Chol-dependent. Similarly, 7KC caused the phasor plot data to move along the chord towards the pure disordered phase. This represents a conversion of areas of ordered phase to a disordered state, rather than the generation of any intermediate state or an effect on disordered regions themselves. Hence, 7KC is a potent agent to modulate raft coverage, lowering the ordered-phase-derived fluorescence to 23±11% ( n =6 cells) of the total signal without affecting cell viability [31] . Association with ordered phases retards LAT diffusion The existence and abundance of ordered lipid domains raises the question of whether they modulate protein behaviour. Hence, we simultaneously recorded membrane order from Laurdan’s emission profile and protein diffusion using fluorescence correlation spectroscopy (FCS) ( Fig. 3 ). We selected the transmembrane protein LAT as our protein of interest because its two palmitoylation sites are thought to target it to ordered membranes [32] . This (to our knowledge, first) quantitative correlation between membrane order and protein diffusion showed a statistically significant negative correlation for wild-type LAT (WT LAT, −0.45, P <0.0063) but not for a palmitoylation-deficient mutant (CS LAT; −0.09, P >0.05; Fig. 3a ). These correlations were not due to manipulations of the local membrane order by the LAT variants as the mean GP values in the plasma membrane remain unchanged at 0.41±0.09 and 0.41±0.04 ( P >0.05) for cells expressing WT and CS LAT, respectively ( Supplementary Fig. S4 ). The data therefore indicate that for WT LAT, diffusion is significantly hindered in higher-order membrane regions. The interactions of LAT with raft domains are facilitated by the palmitoylation groups because CS LAT diffusion was insensitive to membrane order ( Fig. 3a ). Importantly, interactions with sub-resolution lipid domains also influences ensemble measurements, as demonstrated by fluorescence recovery after photobleaching of WT LAT and CS LAT ( Supplementary Fig. S5 ). 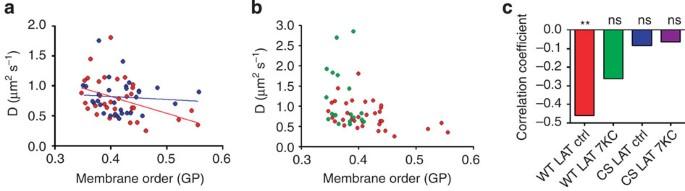Figure 3: Correlation between membrane order and protein diffusion. HeLa cells were transfected with WT LAT or palmitoylation-deficient CS LAT, both fused to mCherry, labelled with Laurdan and data recorded from live cells at room temperature. Pulsed-interleaved excitation was used to alternatively excite Laurdan and mCherry. Laurdan’s emission profile was recorded in two channels, from which the membrane order was quantified as generalized polarization (GP) values. GP values range from −1 to +1, indicating low to high membrane order. TCSPC data of mCherry was used for FCS measurements, from which diffusion coefficients were extracted. (a) Correlation of the diffusion coefficient and membrane order for WT LAT (red) and CS LAT (blue). (b) HeLa cells were treated with 7KC (25 μM for 30 min) to reduce the abundance of ordered phases. Correlation of the diffusion coefficient and membrane order for WT LAT in untreated (red) and 7KC-enriched cells (green). Ina,b, each point represents one FCS/GP measurement. Lines represent linear least-squares-fit trend lines. (c) Correlation coefficients for WT LAT and CS LAT in untreated and 7KC-treated cells (**P<0.01; ns,P>0.05;n=20–30). Figure 3: Correlation between membrane order and protein diffusion. HeLa cells were transfected with WT LAT or palmitoylation-deficient CS LAT, both fused to mCherry, labelled with Laurdan and data recorded from live cells at room temperature. Pulsed-interleaved excitation was used to alternatively excite Laurdan and mCherry. Laurdan’s emission profile was recorded in two channels, from which the membrane order was quantified as generalized polarization (GP) values. GP values range from −1 to +1, indicating low to high membrane order. TCSPC data of mCherry was used for FCS measurements, from which diffusion coefficients were extracted. ( a ) Correlation of the diffusion coefficient and membrane order for WT LAT (red) and CS LAT (blue). ( b ) HeLa cells were treated with 7KC (25 μM for 30 min) to reduce the abundance of ordered phases. Correlation of the diffusion coefficient and membrane order for WT LAT in untreated (red) and 7KC-enriched cells (green). In a , b , each point represents one FCS/GP measurement. Lines represent linear least-squares-fit trend lines. ( c ) Correlation coefficients for WT LAT and CS LAT in untreated and 7KC-treated cells (** P <0.01; ns, P >0.05; n =20–30). Full size image To show that the diffusion of WT LAT is indeed dependent on membrane order, we manipulated the abundance of higher-order membrane domains by treating cells with 7KC. As anticipated, 7KC treatment resulted in an increase in the diffusion coefficient of WT LAT (from 0.78±0.33 to 1.18±0.20 μm 2 s −1 , P <0.05) but not for CS LAT ( P >0.05). The loss of ordered domains by 7KC treatment also reduced the correlation coefficient for both WT LAT and CS LAT ( Fig. 3b ), so that there is no significant difference in diffusion coefficient between WT LAT and CS LAT ( P >0.05), and neither of the two diffusion coefficients are dependent on the degree of membrane order. These data therefore indicate that higher-order lipid domains retard WT LAT diffusion. Lipid phases regulate LAT clustering To determine whether the modulation of diffusion caused by lipid domains is functionally important, we assessed LAT distributions and quantified the degree of clustering into meso-scaled domains that facilitate signal transduction [17] . We employed super-resolution photoactivated localization microscopy (PALM) to obtain molecular coordinates of WT LAT and CS LAT with <50 nm precision, removed repeatedly excited molecules ( Supplementary Fig. S6 ) and calculated quantitative cluster maps ( Fig. 4a ) as previously performed [11] , [33] . The Ripley’s K -function curves ( Fig. 4b ) and the corresponding cluster parameters ( Fig. 4d ) show significant clustering above a random distribution in all tested conditions. WT LAT was significantly less clustered than CS LAT in untreated cells or when compared with WT LAT in 7KC-treated cells. Hence, contrary to the notion that rafts are assembly platforms, the interaction of WT LAT with ordered lipid domains not only retards its diffusion but also limits the degree of meso-scaled clustering. In contrast to WT LAT, 7KC treatment decreased clustering of CS LAT. This behaviour can be explained if the accessible membrane area is considered because CS LAT may be forced to aggregate in the low-abundance disordered phases in untreated cells, which expand upon 7KC treatment. In summary, we propose a membrane model where the majority of plasma membrane is covered by ordered membranes that differentially regulate the diffusion and clustering of LAT variants ( Fig. 5 ). 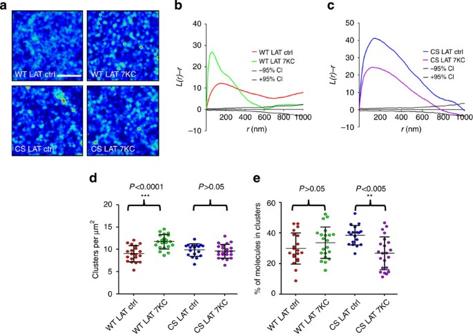Figure 4: Super-resolution PALM imaging and molecular analysis of LAT clustering. HeLa cells were transfected with WT LAT or CS LAT, both fused to the photo-switchable fluorescent protein mEos2, enriched in 7KC or left untreated (Ctrl) and fixed. PALM images were obtained under total internal reflection fluorescence illumination and repeatedly excited fluorophores and molecules, with a localization precision worse than 50 nm removed from further analysis. (a) Quantitative, pseudo-coloured cluster maps generated from Getis and Franklin’s analysis of single-molecule point-pattern data of WT LAT and CS LAT in control and 7KC-treated HeLa cells. Red areas indicate enhanced local molecular density. Scale bar, 1 μm. (b,c). Representative Ripley’sK-function plots for WT LAT (b) in untreated (red line) and 7KC-enriched cells (green line) and for CS LAT (c) in untreated (blue line) and 7KC-enriched cells (purple line), quantifying the level of clustering (L(r)-r). The 95% confidence intervals (black lines) were obtained from 100 simulations of random distributions. (d,e) Density of LAT clusters (d) and percentage of LAT molecules residing in clusters (e) were obtained from thresholded cluster maps. Each symbol represents one 3 × 3 μm2image region. Regions were selected from seven cells per condition; horizontal bars and error bars show mean and s.d., respectively (**P<0.05; ***P<0.0001). Figure 4: Super-resolution PALM imaging and molecular analysis of LAT clustering. HeLa cells were transfected with WT LAT or CS LAT, both fused to the photo-switchable fluorescent protein mEos2, enriched in 7KC or left untreated (Ctrl) and fixed. PALM images were obtained under total internal reflection fluorescence illumination and repeatedly excited fluorophores and molecules, with a localization precision worse than 50 nm removed from further analysis. ( a ) Quantitative, pseudo-coloured cluster maps generated from Getis and Franklin’s analysis of single-molecule point-pattern data of WT LAT and CS LAT in control and 7KC-treated HeLa cells. Red areas indicate enhanced local molecular density. Scale bar, 1 μm. ( b , c ). Representative Ripley’s K -function plots for WT LAT ( b ) in untreated (red line) and 7KC-enriched cells (green line) and for CS LAT ( c ) in untreated (blue line) and 7KC-enriched cells (purple line), quantifying the level of clustering ( L(r)-r ). The 95% confidence intervals (black lines) were obtained from 100 simulations of random distributions. ( d , e ) Density of LAT clusters ( d ) and percentage of LAT molecules residing in clusters ( e ) were obtained from thresholded cluster maps. Each symbol represents one 3 × 3 μm 2 image region. Regions were selected from seven cells per condition; horizontal bars and error bars show mean and s.d., respectively (** P <0.05; *** P <0.0001). 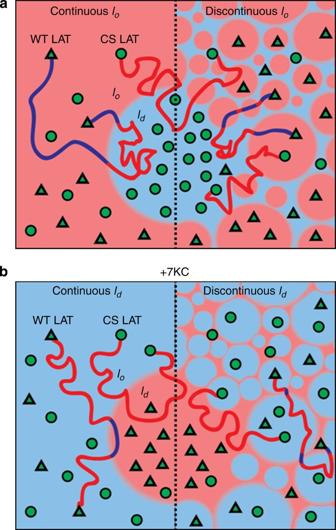Figure 5: Proposed model of membrane organization. (a) Membrane regions of high lipid order that correspond to liquid-ordered phases in model membranes (lo, regions shaded in pink) cover 76±6% of the plasma membrane in HeLa cells. There are two possible geometries; either the liquid-ordered phase percolates through disordered-phase domains (ld, regions shaded in light blue) (left) or thelodomains exist of various size that are densely packed (right) within a percolatingldphase. WT LAT (triangles) can cross domain boundaries and diffuses slower (blue traces) in ordered membranes and faster (red traces) in disordered membranes. If CS LAT crosses domain boundaries, the lipid environment has no effect on its diffusion. There are two mechanisms, which are not mutually exclusive that can account for the greater degree of clustering of CS LAT compared with WT LAT. CS LAT may be confined to smalllddomains; or the faster average diffusion of CS LAT increases the collision probability with other molecules and, hence, the propensity for self-association. (b) After 7KC enrichment,ldphases dominate, accelerating WT LAT diffusion as these molecules spend on average less time inlodomains, whereas having no effect on CS LAT diffusion. CS LAT clustering is decreased as it is no longer confined in smalllddomains, and WT LAT clustering is increased due to increased confinement and faster diffusion. Full size image Figure 5: Proposed model of membrane organization. ( a ) Membrane regions of high lipid order that correspond to liquid-ordered phases in model membranes ( l o , regions shaded in pink) cover 76±6% of the plasma membrane in HeLa cells. There are two possible geometries; either the liquid-ordered phase percolates through disordered-phase domains ( l d , regions shaded in light blue) (left) or the l o domains exist of various size that are densely packed (right) within a percolating l d phase. WT LAT (triangles) can cross domain boundaries and diffuses slower (blue traces) in ordered membranes and faster (red traces) in disordered membranes. If CS LAT crosses domain boundaries, the lipid environment has no effect on its diffusion. There are two mechanisms, which are not mutually exclusive that can account for the greater degree of clustering of CS LAT compared with WT LAT. CS LAT may be confined to small l d domains; or the faster average diffusion of CS LAT increases the collision probability with other molecules and, hence, the propensity for self-association. ( b ) After 7KC enrichment, l d phases dominate, accelerating WT LAT diffusion as these molecules spend on average less time in l o domains, whereas having no effect on CS LAT diffusion. CS LAT clustering is decreased as it is no longer confined in small l d domains, and WT LAT clustering is increased due to increased confinement and faster diffusion. Full size image We demonstrated that the phasor approach to FLIM data analysis [25] , [26] is able to unmix the signals from ordered and disordered phases in cellular membranes that were stained with Laurdan or di-4-ANEPPDHQ. This method has several advantages over other approaches that can also be used to measure membrane order. Unlike the quantification of the generalized polarization (GP) [22] , the phasor approach can distinguish between a mixture of immiscible phases and a homogenous environment with intermediate order. And unlike spectral unmixing or fitting multi-exponential FLIM data, it requires no a priori knowledge of the number of components that need to be unmixed [26] . In other words, in our analysis, there is no assumption that the membrane is a two-component system. However, there are also limitations that this approach cannot overcome. For example, the phasor analysis does not provide information about domain size and distribution, other than that the domains are smaller than the diffraction limit; and hence, the geometry of a two-component system is not known. In addition, acquisition speed for FLIM data is generally slower than for spectral imaging, making it difficult to study dynamic processes or measure the lifespan of domains and fluctuations. It should also be noted that phase separation reported by lipid-packing sensing dyes does not exclude the possibilities of domains that are formed by other principles such as membrane charges [34] , [35] and electrostatic interactions [36] , [37] . Our data clearly demonstrate that sub-resolution phases exist in live cell membranes. These phases correspond to the classical liquid-ordered and -disordered phases that have been observed in artificial membrane systems. Contrary to the classical lipid raft hypothesis, we found that the majority of the plasma membrane resides in the liquid-ordered phase. Similar observations have been made previously using phase-partitioning dyes in vesicles composed of plasma membrane lipids [30] . The raft-majority membrane may constitute a dense array of ordered-phase domains, such as proposed for rabbit red blood cells, in a recent study that employed fluorescence fluctuation analysis of Laurdan [28] , or a percolating raft phase containing disordered-phase domains ( Fig. 5a ) as suggested for the apical membranes of polarized epithelial cells [29] and CHO cells [28] . It is possible that the plasma membrane of cells can switch between these configurations based on temperature or activation status, for example, during signalling. This would constitute a novel compartmentalization process that may not be dependent on large-scale changes in the lipid composition but more importantly, would be reversible. For example, membrane condensation was observed at T-cell activation sites [21] and immunological synapses [38] , and it is such high membrane order that supports the formation of T-cell receptor microclusters and T-cell activation [31] . Hence, it is possible that high membrane order at these sites is caused by the delivery of sub-synaptic vesicles [33] , [39] , an increase in coverage of ordered phases in the plasma membrane or large-scale lipid-phase separation. The latter is more unlikely because T-cell activation sites are regions of highly dynamic actomyosin activity, which may cause the ordered phase to fracture into discreet domains in an ‘active’ energy-dependent process [40] . More detailed mapping of the coverage of lipid phases and/or domain sizes, possibly in conjunction with stimulated emission depletion [15] and Laurdan GP fluctuation analysis [28] , may reveal a more complex regulation of lipid domain geometries than previously thought. One of the central tenets of the lipid raft hypothesis is the ability of microdomains to cluster raft-favouring proteins, and thereby facilitate protein–protein interactions. We observed that ordered lipid domains are not only the dominant phase in the plasma membrane, but that association with these domains retards diffusion and is likely to randomize the distributions of these proteins. In the case of LAT, the protein that was associated with the dominant phase, that is, WT LAT in non-treated cells and CS LAT in 7KC-treated cells, was more randomly distributed compared with its counterpart in the minor phase ( Fig. 5 ). It is possible that the higher clustering observed for the faster diffusing species, for example, CS LAT in control cells, may be in part the result of fewer collisions between the molecules. If association with dominant versus minor phase is a general rule for protein distribution, it will be important to map the driving forces for phase coverage and phase association in intact cells. In the case of T-cell activation, phase partitioning of signalling proteins and the geometry of lipid domains may hold the key to which receptor interactions are prevented or ‘inhibited’ in resting cells and ‘allowed’ in activated cells, simply through spatial reorganization [17] . It is apparent that the abundance or surface coverage of ordered lipid phases we measured does not match the abundance of protein domains that have been reported previously, which range from nano-scaled complexes [12] to meso-scaled clusters [11] , [33] and islands [17] . Although lipid domains contribute to the regulation of protein clustering (see effect of 7KC treatment in Fig. 4 ), additional factors including weak and strong protein–protein interactions [41] , confinement by the actin cytoskeleton [18] and actomyosin driven flow [40] must also be responsible for protein distributions. The combinations of various mechanisms of membrane compartmentalization may yield a diverse range of membrane structures scaling from nano-scaled lipid and protein complexes [12] , [41] to meso-scaled domains and long-range networks [42] . It is also possible that these membrane-organizing forces are interlinked, so that protein networks, for example, may position lipid phases, which in turn regulate protein diffusion and localization. It is equally possible that other compartmentalization mechanisms facilitate the switch between dense array of lipid domains of various sizes and a percolating ordered phase that is discussed above. In summary, we propose that lipid phases ought to be integrated into a holistic view of membrane organization [43] , for which the phasor analysis of FLIM data of membrane–order sensing dyes provides an experimental basis. Sample preparation HeLa cells were cultured in DMEM media (Gibco) in 10% fetal calf serum at 37 °C and 5% humidity. For FCS, cells were transfected with mCherry fusion proteins of WT LAT or a non-palmitoylated LAT mutant (CS LAT) using Lipofectamine LTX (Invitrogen) and imaged 24 h after transfection. Cells were left untreated or treated with either 25 μM 7KC complexed to mβCD for 30 min at 37 °C or with unloaded 5 mM mβCD for 20 min. For PALM, cells were transfected with human WT LAT-mEOS2 and the CS-mutant of LAT fused to mEOS2 ( [33] ). For FLIM and FCS measurements, cells were stained with 5 mM Laurdan or di-4-ANEPPDHQ (both Invitrogen) by adding 2 μl of a 5 mM stock in dimethylsulphoxide (DMSO) to the media [22] . For PALM, cells were fixed with 4% paraformaldehyde for 30 min at 37 °C. Lipid bilayers were formed by drying mixtures of DOPC, SM and Chol in chloroform, followed by hydration in PBS in a sonicating water bath at 37 °C. FLIM measurements and phasor plotting FLIM measurements were acquired using a Picoquant Microtime200 inverted confocal microscope with a X63 1.2 numerical aperture (NA) water-immersion objective. Laurdan was excited using a 405 nm diode laser at a repetition rate of 40 MHz. Fluorescence was detected though a 430 nm long-pass filter using a single-photon avalanche diode (PDM, MPD, Bolzano, Italy) and PicoHarp300 TCSPC electronics. Fluorescein solution was used as a calibration sample. Data were imported into Globals Software (SimFCS 2.0 LFD; Irvine, CA) and displayed as a phasor plot (plot of S against g ) as previously described [26] by applying the transformations: Where ω=2πf and f is the laser repetition rate, and I(t) is the fluorescence intensity at time t . On a plot of g against S (a phasor plot), a single-exponential decay lies on a semicircle centred on ( g , S )=(0.5,0) and with radius 0.5. Double-exponential decays lie on a chord connecting the two single-exponential positions. Details on FCS setup and fitting FCS measurements were acquired using a Picoquant Microtime200 confocal microscope equipped with a X63 1.2 NA water-immersion objective. Laurdan was excited by a diode laser operating at 405 nm. Laurdan Fluorescence was separated into 2-channels using a 458 nm long-pass dichroic followed by band-pass filters. Intensity values in each channel were then used to calculate the Laurdan generalized polarization (GP) value using equation 3: Where I represents the intensity in each channel and G is a calibration factor calculated using equation 4: Where GP mes is the measured GP value of Laurdan in DMSO and GP ref is a reference value for Laurdan in DMSO, defined to be GP ref =0.207. 405 and 532 nm lasers for mCherry excitation were used in a pulsed-interleaved excitation configuration at a total excitation rate of 40 MHz. This eliminated cross-talk between the Laurdan and mCherry channels caused by spectral bleedthrough. mCherry fluorescence was also spectrally separated from the Laurdan signal using a 580-nm short-pass dichroic and a 581–653 nm band-pass filter. Fluorescence lifetime correlation spectroscopy of the time-correlated single-photon counting data was used to weight photons according to their arrival time to eliminate correlations due to after-pulsing from the detector. After correction, FCS curves were fitted to a two-dimensional Brownian diffusion model, and the diffusion coefficient was extracted using Picoquant SymPhoTime software. Rhodamine in water at room temperature was used as an FCS calibration standard. PALM and cluster analysis PALM images of WT LAT-mEos2 and CS LAT-mEos2 were acquired on a Zeiss Elyra PS1 microscope with a X100 1.46 NA oil-immersion objective. Photoconversion of mEOS2 was achieved by irradiation with a 405 nm laser. The converted form was excited at 561 nm. A total of 15,000 frames with an exposure time of 30 ms were recorded on an electron multiplying CCD camera (iXon DU-897D; Andor). Recorded images were analysed using Zen 2010D (Carl Zeiss MicoImaging). The software fits a two-dimensional Gaussian distribution to each detected event, thereby determining the centre of each point spread function (PSF) along with the localization precision. Sample drift during the acquisition was corrected for by tracking several immobile, 100 nm gold fiducial markers. The data were filtered to remove molecules with localization precisions >50 nm and molecules that were repeatedly excited during the acquisition process, as previously described [44] , [45] , [46] ( Supplementary Fig. S6 ). Spatial point patterns were analysed using Ripley’s K-function [47] , calculated using SpPack [48] as equation 5: Here, n is the number of points contained in a field-of-view of area A (a 3 × 3 μm 2 square area). d ij is the distance between two points i and j and r is the analysed spatial scale. This function is a measure of the number of points, j , encircled within concentric circles of radius r centred on each point i . The K-function scales with circle area, and for a completely spatially random (CSR) case, scales linearly with area. It is therefore transformed into the L-function, such that scaling is linear with radius, r using equation 6: For a CSR case, it follows that L(r)=r at all radii. A plot of L(r) − r versus r , therefore has L(r)−r=zero at all r for a CSR distribution. If more points have been encircled at a given radius than would have been expected of a random distribution, L(r)−r is positive, and the points are clustered. The 99% confidence intervals for cluster detection were calculated by simulating 100 CSR distributions with the same average molecular density as the data. Edge effects in the analysis were corrected for by weighting edge points accordingly. To construct cluster maps, we performed Getis and Franklin’s analysis where the value of L(r) is calculated for each point, j , individually at a specific spatial scale, here, 50 nm. A quantitative, pseudo-coloured cluster map is then interpolated on a 10 nm resolution grid. This map was then thresholded at a value of L (50)=80 to generate a binary cluster map from which clustering parameters (such as number of clusters, cluster size, shape, number of molecules per cluster and so on) could then be extracted [33] . How to cite this article: Owen, D.M. Sub-resolution lipid domains exist in the plasma membrane and regulate protein diffusion and distribution. Nat. Commun. 3:1256 doi: 10.1038/ncomms2273 (2012).